Fragile X mental retardation protein stimulates ribonucleoprotein assembly of influenza A virus The ribonucleoprotein (RNP) of the influenza A virus is responsible for the transcription and replication of viral RNA in the nucleus. These processes require interplay between host factors and RNP components. Here, we report that the Fragile X mental retardation protein (FMRP) targets influenza virus RNA synthesis machinery and facilitates virus replication both in cell culture and in mice. We demonstrate that FMRP transiently associates with viral RNP and stimulates viral RNP assembly through RNA-mediated interaction with the nucleoprotein. Furthermore, the KH2 domain of FMRP mediates its association with the nucleoprotein. A point mutation (I304N) in the KH2 domain, identified from a Fragile X syndrome patient, disrupts the FMRP–nucleoprotein association and abolishes the ability of FMRP to participate in viral RNP assembly. We conclude that FMRP is a critical host factor used by influenza viruses to facilitate viral RNP assembly. Our observation reveals a mechanism of influenza virus RNA synthesis and provides insights into FMRP functions. The replication of a virus relies on arrays of virus–host interactions to support each step of the virus life cycle and to allow the virus to subvert host defence. Unlike most RNA viruses, influenza replicates and transcribes its RNA in the nucleus of infected cells rather than in the cytoplasm. The identification of host factors that participate in influenza virus replication is of great interest to provide a better understanding of the mechanisms of the viral life cycle and for the discovery of potential targets for antiviral therapy [1] , [2] , [3] , [4] , [5] , [6] . The genome of influenza A viruses is composed of eight single-stranded, negative-sense RNAs, which encode at least 10 proteins. Each RNA segment is encapsidated by multiple copies of the viral nucleoprotein (NP), and is associated with RNA-dependent RNA polymerase (RdRp), forming a viral ribonucleoprotein complex (vRNP) [7] . The purified virion RNPs appear as flexible, closed, superhelical structures under electron microscopy [8] . The vRNP is an independent functional unit catalysing viral RNA transcription (vRNA→mRNA) and replication (vRNA→cRNA→vRNA) in the nucleus of infected cells [9] . Within the vRNPs, RdRp, a heterotrimeric complex consisting of three subunits PB1, PB2 and PA, is responsible for the synthesis of three species of viral RNAs (vRNA, mRNA and cRNA) [9] , [10] . NP, associated with both viral RNA and RdRp, is a key structural determinant of vRNP [11] , [12] . The efficiency of viral RNA synthesis, which is critical for virus multiplication and pathogenicity, is dependent on the RNP assembly and RdRp activity [10] , [13] , [14] , [15] . However, mechanisms of RNP assembly remain largely unknown. An assembly model has been proposed for the RdRp in which the assembly may occur between the individually transported PB1-PA dimer and PB2 monomer in the nucleus [16] , [17] , [18] . However, how NP assembles with RdRp and viral RNA in the nucleus is unclear. Using a cellular transcription profiling-based RNAi screen, we have identified here that the Fragile X mental retardation protein (FMRP) acts as a positive regulator of influenza virus replication. FMRP is an RNA-binding protein harbouring two KH-type (KH1 and KH2)-binding domains and an RGG-type RNA-binding domain. It has the ability to bind to different mRNAs/RNAs [19] , [20] . In addition, FMRP carries functional nuclear localization signals (NLSs) and nuclear export signals and is believed to shuttle between the cytoplasm and nucleus [21] , [22] . FMRP is implicated in intracellular RNA transport and regulation of translation at synapses [23] . The absence or specific mutation(s) of FMRP leads to Fragile X syndrome (FXS) [24] . FXS is the most common cause of inherited mental retardation and autism [25] . A point mutation I304N in the KH2 domain of FMRP is associated with the Fragile X syndrome, indicating a key role of the KH2 domain in FMRP functions [26] . It remains unclear how RNA binding to FMRP is implicated in FXS [25] . In this report, we found that FMRP is required for influenza virus replication both in cell culture and in mice. We further show that FMRP interacts with NP of influenza A viruses in an RNA-dependent manner. FMRP transiently associates with viral RNPs and stimulates viral RNP assembly in a manner that is dependent on its KH2 domain and the I304 residue. FMRP knockdown leads to nuclear retention of viral RNP components. These data expand our knowledge on influenza virus RNP assembly and FMRP functions. Screen of host factors involved in influenza virus infection In the present study, we combined cellular transcriptional profiling with a small interfering RNA (siRNA) screen to identify host factors involved in influenza virus replication. A549 human lung epithelial cells were infected with influenza A/PR/8/34 (PR8) virus and harvested at 4, 12, 24 and 48 h post infection (h.p.i.). Total RNA was analysed by microarray. On the basis of a threshold of fold change ≥2.0 and a P -value <0.01 (Student’s t -test), 300 host genes were considered significantly upregulated. We then conducted an siRNA screen using a library against these upregulated genes. For this purpose, A549 cells were transfected with siRNAs, infected with PR8 virus and subjected to immunofluorescence analysis using an NP-specific antibody ( Fig. 1a ). Using a twofold change as a threshold, the screen revealed 41 host factors as potential positive regulators and 11 host factors as negative regulators of influenza virus replication. 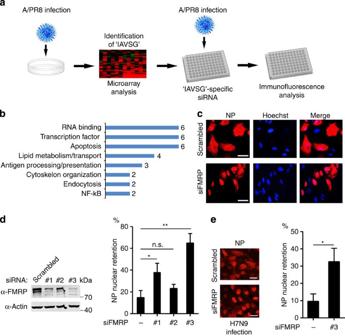Figure 1: Cellular transcriptional profiling-based siRNA screen for host factors involved in influenza A virus replication. (a) Illustration of the siRNA screen procedures. IAVSG, influenza A virus-stimulated genes. (b) Functional classification of identified genes. Numbers of identified genes per category were indicated. (c) Immunofluorescence images of cells treated with control or FMRP-specific siRNA and infected with PR8 virus. Scale bar, 20 μm. (d) The reduction in the FMRP protein level correlated with the extent of NP nuclear accumulation. A549 cells were treated with control or three individual FMRP-specific siRNAs. After 48 h, cells were lysed and subjected to western blot analyses (left), or were infected with PR8 viruses (right, see alsoSupplementary Fig. 1f), followed by immunofluorescence analysis. Quantitative analyses were calculated by ratios of NP nuclear-retained cells/total infected cells (mean±s.d. of three independent experiments, *P<0.05, **P<0.01, n.s., not significant, two-tailed Student’st-test). (e) FMRP knockdown resulted in NP nuclear retention in cells infected with H7N9 influenza A virus. A549 cells were treated with the indicated siRNA, infected with H7N9 influenza A virus (A/Anhui/1/2013) at an MOI of 0.1 for 9 h, and were subjected to the immunofluorescence assay and quantitatively analysed (mean±s.d. of three independent experiments, *P<0.05, two-tailed Student’st-test). Scale bar, 20 μm. Forty of the fifty-two genes have not been previously reported ( Table 1 ; Supplementary Data 1–3 ). Functional classification analysis revealed that these host factors were enriched in gene categories associated with RNA binding, transcription and apoptosis, which may be involved in different stages of the influenza virus life cycle ( Fig. 1b ; Supplementary Data 4 ). Figure 1: Cellular transcriptional profiling-based siRNA screen for host factors involved in influenza A virus replication. ( a ) Illustration of the siRNA screen procedures. IAVSG, influenza A virus-stimulated genes. ( b ) Functional classification of identified genes. Numbers of identified genes per category were indicated. ( c ) Immunofluorescence images of cells treated with control or FMRP-specific siRNA and infected with PR8 virus. Scale bar, 20 μm. ( d ) The reduction in the FMRP protein level correlated with the extent of NP nuclear accumulation. A549 cells were treated with control or three individual FMRP-specific siRNAs. After 48 h, cells were lysed and subjected to western blot analyses (left), or were infected with PR8 viruses (right, see also Supplementary Fig. 1f ), followed by immunofluorescence analysis. Quantitative analyses were calculated by ratios of NP nuclear-retained cells/total infected cells (mean±s.d. of three independent experiments, * P <0.05, ** P <0.01, n.s., not significant, two-tailed Student’s t -test). ( e ) FMRP knockdown resulted in NP nuclear retention in cells infected with H7N9 influenza A virus. A549 cells were treated with the indicated siRNA, infected with H7N9 influenza A virus (A/Anhui/1/2013) at an MOI of 0.1 for 9 h, and were subjected to the immunofluorescence assay and quantitatively analysed (mean±s.d. of three independent experiments, * P <0.05, two-tailed Student’s t -test). Scale bar, 20 μm. Full size image Table 1 Host genes involved in influenza A virus replication. Full size table Interestingly, we observed that knockdown of the FMR1 gene in A549 cells infected with PR8 virus showed nuclear accumulation of NP in the immunostaining assay ( Fig. 1c ). This phenotype was confirmed by confocal microscopy and subcellular fractionation assays ( Supplementary Fig. 1a–d ). In addition, we tested six individual siRNAs ( Supplementary Fig. 1e ) and then used three of them to knock down FMRP. This revealed that the reduction of the FMRP protein level correlated with the extent of NP nuclear retention ( Fig. 1d ; Supplementary Fig. 1f ). Furthermore, we confirmed the phenotype with a novel avian-origin H7N9 influenza virus strain (A/Anhui/1/2013) ( Fig. 1e ), suggesting that FMRP may play a general role among influenza A viruses. Finally, we monitored the dynamics of NP trafficking during viral infection and found that NP nuclear import was unaffected, while its nuclear export was impeded in the FMRP-knockdown cells ( Supplementary Fig. 2 ). Together, these results suggest that FMRP is associated with influenza A virus NP/RNP nuclear export. FMRP is required for influenza A virus replication We next examined the effect of FMRP in influenza A virus replication. FMRP-stable knockdown 293T cells and control cells ( Fig. 2a ) were infected with influenza A/WSN/33 (WSN) virus, and then viral supernatants were harvested and subjected to TCID 50 analyses on MDCK cells. This assay revealed that viral growth was remarkably reduced in the FMRP-knockdown cells by about 1 log ( Fig. 2b ). In contrast, when the FMRP-knockdown and control cell lines were infected with the Newcastle disease virus, no significant differences in virus growth were detected ( Supplementary Fig. 3a ). Because influenza viruses are susceptible to host interferons (IFNs), we examined the effect of FMRP on IFN activation. This revealed that FMRP did not affect IFN-β promoter activity ( Supplementary Fig. 3b,c ). Together, these results suggest that FMRP supports influenza virus replication in cell culture. To investigate whether FMRP also supports influenza virus replication in vivo , we infected wild-type (WT) and FMRP-knockout (FMRP −/− ) mice with PR8. By histopathological analysis, we found that lungs of WT mice showed more severe injury and inflammation compared with those of FMRP −/− mice ( Fig. 2c,d ). Further, immunohistochemistry staining of NP revealed that viral antigen was reduced in FMRP −/− mice ( Fig. 2e ). Consistently, virus titres in the lungs of FMRP −/− mice were decreased by ~1 log compared with WT ( Fig. 2f ; Supplementary Fig. 4 ). The infected WT mice underwent increased weight loss compared with FMRP −/− mice ( Fig. 2g ; Supplementary Tables 1 and 2 ). It should be noted that some of the WT and FMRP −/− mice (FVB strain background) underwent infection-caused growth arrest rather than significant weight loss ( Supplementary Tables 1 and 2 ). This weight-loss profile was consistent with the previously published data reporting that compared with other mouse strains (for example, C57BL/6 or BALB/c) FVB mice were the least affected by the weight loss on influenza PR8 virus infection [27] . Moreover, while ~80% of the WT mice succumbed to infection, ~65% of the FMRP −/− mice survived ( Fig. 2h ). Taken together, these data highlight that FMRP is required for efficient influenza A virus replication in vitro and in vivo . 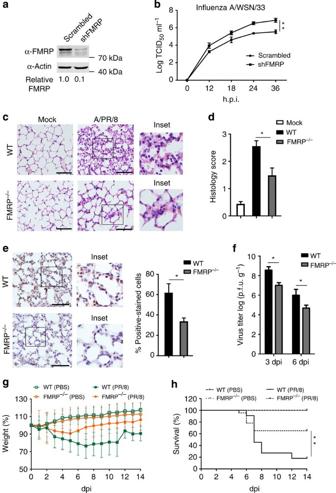Figure 2: Knockdown of FMRP impairs influenza virus replication in cell culture and in mice. (a) Protein levels of FMRP in FMRP-stable knockdown 293T cells (shFMRP) or control cells (scrambled). (b) Knockdown of FMRP specifically attenuates influenza virus replication in cell culture. shFMRP cells or control cells were infected with influenza A/WSN/33 (WSN) virus (MOI=0.01); supernatants were then harvested at the indicated time points and subjected to TCID50assays (mean±s.d. of three independent experiments, **P<0.01, two-tailed Student’st-test). (c) H&E staining of the lungs of WT and FMRP−/−mice infected with 104TCID50of PR8 virus on day 3 p.i. (magnification × 400). Scale bar, 100 μm. (d) Histological scoring of H&E-stained lung sections as shown in (c) (mean±s.d., *P<0.05, two-tailed Student’st-test). WT (n=3), FMRP−/−(n=3) and WT mock-infected (n=3). (e) Left: immunohistochemical detection of NP in the lungs of WT or FMRP−/−mice infected with PR8 virus on day 3 p.i. (magnification × 400). Scale bar, 100 μm. Right: statistical analysis of positively immunostained cells (mean±s.d.,n=3, *P<0.05, two-tailed Student’st-test). (f) Viral lung titres of WT and FMRP−/−mice on days 3 and 6 p.i. (mean±s.d.,n=3, *P<0.05, two-tailed Student’st-test, see alsoSupplementary Fig. 4). (g,h) Infected WT (n=11) and FMRP−/−mice (n=23) were monitored for 14 days for weight loss (g) and survival (h). Control groups received PBS only (WT,n=4 and FMRP−/−,n=4). Survival in FMRP−/−mice was significantly enhanced compared with WT animals (mean±s.d., **P<0.01, two-tailed Student’st-test). None of the PBS-inoculated control groups lost weight and all survived. Data are representative of two independent experiments. Figure 2: Knockdown of FMRP impairs influenza virus replication in cell culture and in mice. ( a ) Protein levels of FMRP in FMRP-stable knockdown 293T cells (shFMRP) or control cells (scrambled). ( b ) Knockdown of FMRP specifically attenuates influenza virus replication in cell culture. shFMRP cells or control cells were infected with influenza A/WSN/33 (WSN) virus (MOI=0.01); supernatants were then harvested at the indicated time points and subjected to TCID 50 assays (mean±s.d. of three independent experiments, ** P <0.01, two-tailed Student’s t -test). ( c ) H&E staining of the lungs of WT and FMRP −/− mice infected with 10 4 TCID 50 of PR8 virus on day 3 p.i. (magnification × 400). Scale bar, 100 μm. ( d ) Histological scoring of H&E-stained lung sections as shown in ( c ) (mean±s.d., * P <0.05, two-tailed Student’s t -test). WT ( n =3), FMRP −/− ( n =3) and WT mock-infected ( n =3). ( e ) Left: immunohistochemical detection of NP in the lungs of WT or FMRP −/− mice infected with PR8 virus on day 3 p.i. (magnification × 400). Scale bar, 100 μm. Right: statistical analysis of positively immunostained cells (mean±s.d., n =3, * P <0.05, two-tailed Student’s t -test). ( f ) Viral lung titres of WT and FMRP −/− mice on days 3 and 6 p.i. (mean±s.d., n =3, * P <0.05, two-tailed Student’s t -test, see also Supplementary Fig. 4 ). ( g , h ) Infected WT ( n =11) and FMRP −/− mice ( n =23) were monitored for 14 days for weight loss ( g ) and survival ( h ). Control groups received PBS only (WT, n =4 and FMRP −/− , n =4). Survival in FMRP −/− mice was significantly enhanced compared with WT animals (mean±s.d., ** P <0.01, two-tailed Student’s t -test). None of the PBS-inoculated control groups lost weight and all survived. Data are representative of two independent experiments. Full size image FMRP targets influenza viral RNA synthesis machinery To study the mechanism(s) by which FMRP regulates influenza A virus replication, we first examined the role of FMRP in viral protein and RNA synthesis in infected cells. Western blot analyses of lysates from FMRP-knockdown cells infected with WSN showed reduction of viral NP and PA protein levels at various time points p.i. ( Supplementary Fig. 5a ). Primer extension analysis revealed reduced levels of viral mRNA, cRNA and vRNA of the viral neuraminidase (NA) segment in the FMRP-knockdown cells ( Fig. 3a,b ). To confirm the role of FMRP in viral RNA synthesis, FMRP was also overexpressed on WSN virus infection. This led to about twofold enhanced viral mRNA, cRNA and vRNA syntheses at all time points p.i. ( Fig. 3c,d ). Taken together, these data indicate that FMRP plays a positive role in viral RNA and protein synthesis. 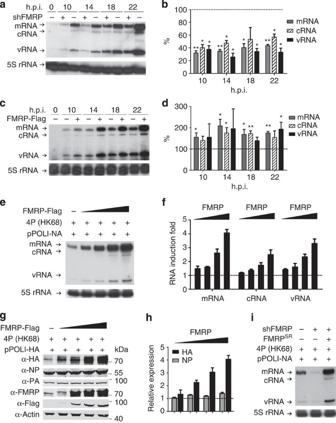Figure 3: FMRP targets influenza virus RNA synthesis machinery. (a) FMRP knockdown reduces influenza virus RNA synthesis. The FMRP-stable knockdown and control 293T cells were infected with WSN virus (MOI=0.01). Total RNAs were harvested at the indicated time points, and the levels of viral vRNA, mRNA and cRNA of the NA segment were detected by primer extension analyses. (b) Statistical analysis of viral RNAs. Values of viral RNAs in (a) were standardized to the 5S rRNA. Values are expressed as a percentage of the control values (mean±s.d. of four independent experiments, *P<0.05, **P<0.01, two-tailed Student’st-test). (c) Overexpression of FMRP stimulates viral RNA synthesis. 293T cells were left untransfected or transfected with FMRP plasmids and then infected with WSN virus (MOI=0.01). Total RNAs were analysed as indicated in (a). (d) Statistical analysis of viral RNAs in (c) (mean±s.d. of four independent experiments, *P<0.05, **P<0.01, two-tailed Student’st-test). (e) FMRP stimulates viral RNA synthesis in an RNP reconstitution system. 293T cells were transfected with influenza A/Hong Kong/1/1968 (H3N2) virus (HK68) RNP reconstitution plasmids, along with an increasing dose of the FMRP plasmids (1, 2, 3 or 4 μg; wedges). Total RNAs were analysed as indicated in (a). (f) Quantitative analysis of viral RNAs in (e). Values of viral RNAs in the FMRP-transfected cells were standardized to the 5S rRNA level and normalized to levels of viral RNAs in cells transfected with a control vector (mean±s.d. of three independent experiments). (g) Overexpression of FMRP does not affect RdRp and NP expression in the RNP reconstitution system. 293T cells were transfected as indicated in (e), except the pPOLI-NA plasmid was replaced with a pPOLI-HA plasmid. Harvested cells were analysed by western blot analyses. (h) Quantitative analysis of protein expression levels in (g) (mean±s.d. of two independent experiments). (i) FMRP specifically regulates viral RNA synthesis in the RNP reconstitution system. The FMRP-stable knockdown or control 293T cells were transfected with the vRNP reconstitution plasmids, together with a control vector or an siRNA-resistant plasmid expressing FMRP (FMRPSR). Total RNAs were analysed as indicated in (a). Figure 3: FMRP targets influenza virus RNA synthesis machinery. ( a ) FMRP knockdown reduces influenza virus RNA synthesis. The FMRP-stable knockdown and control 293T cells were infected with WSN virus (MOI=0.01). Total RNAs were harvested at the indicated time points, and the levels of viral vRNA, mRNA and cRNA of the NA segment were detected by primer extension analyses. ( b ) Statistical analysis of viral RNAs. Values of viral RNAs in ( a ) were standardized to the 5S rRNA. Values are expressed as a percentage of the control values (mean±s.d. of four independent experiments, * P <0.05, ** P <0.01, two-tailed Student’s t -test). ( c ) Overexpression of FMRP stimulates viral RNA synthesis. 293T cells were left untransfected or transfected with FMRP plasmids and then infected with WSN virus (MOI=0.01). Total RNAs were analysed as indicated in ( a ). ( d ) Statistical analysis of viral RNAs in ( c ) (mean±s.d. of four independent experiments, * P <0.05, ** P <0.01, two-tailed Student’s t -test). ( e ) FMRP stimulates viral RNA synthesis in an RNP reconstitution system. 293T cells were transfected with influenza A/Hong Kong/1/1968 (H3N2) virus (HK68) RNP reconstitution plasmids, along with an increasing dose of the FMRP plasmids (1, 2, 3 or 4 μg; wedges). Total RNAs were analysed as indicated in ( a ). ( f ) Quantitative analysis of viral RNAs in ( e ). Values of viral RNAs in the FMRP-transfected cells were standardized to the 5S rRNA level and normalized to levels of viral RNAs in cells transfected with a control vector (mean±s.d. of three independent experiments). ( g ) Overexpression of FMRP does not affect RdRp and NP expression in the RNP reconstitution system. 293T cells were transfected as indicated in ( e ), except the pPOLI-NA plasmid was replaced with a pPOLI-HA plasmid. Harvested cells were analysed by western blot analyses. ( h ) Quantitative analysis of protein expression levels in ( g ) (mean±s.d. of two independent experiments). ( i ) FMRP specifically regulates viral RNA synthesis in the RNP reconstitution system. The FMRP-stable knockdown or control 293T cells were transfected with the vRNP reconstitution plasmids, together with a control vector or an siRNA-resistant plasmid expressing FMRP (FMRP SR ). Total RNAs were analysed as indicated in ( a ). Full size image FMRP has been suggested to play a role in the regulation of translation of specific target mRNAs [23] . We therefore speculated that the positive role of FMRP in regulating influenza virus RNA/protein synthesis may result from its direct upregulation of viral RNA polymerase translation. Alternatively, FMRP may directly stimulate viral RNA synthesis. To dissect these two possible mechanisms, we then examined the effect of FMRP overexpression on viral RNA synthesis in an RNP reconstitution system derived from the influenza A/Hong Kong/1/1968 (H3N2) virus (HK68), in which 293T cells were transiently transfected with either an empty vector or with increasing amounts of the FMRP expression plasmid, together with plasmids encoding PA, PB1, PB2 and NP, as well as a Pol I-driven RNA expression plasmid encoding the NA vRNA segment, forming a minimal viral RNA synthesis unit—the RNP. In this system, the four proteins (PB1, PB2, PA and NP) are constantly produced by the four Pol II-driven expression plasmids. Thus, this approach allows us to examine the specific effect of FMRP on viral RNA transcription and replication ( Supplementary Fig. 5b ). Our results indicate that the levels of all three species of RNAs transcribed by viral RNA polymerase from the input NA vRNA segment are increased with increasing amounts of FMRP expressed ( Fig. 3e,f ), indicating that FMRP stimulates viral RNA synthesis in a dose-dependent manner. To exclude the possibility that the stimulation of viral RNA synthesis by FMRP overexpression may be caused by increased levels of RdRp and/or NP, we further examined the protein levels in the RNP reconstitution system on FMRP overexpression. For this purpose, we replaced the RNA expression plasmid carrying the NA segment with a plasmid carrying a hemagglutinin (HA) segment in the RNP reconstitution system, and examined the levels of HA together with the level of PA and NP by western blot analysis. As expected and consistent with the RNA levels detected, the level of the HA protein also increased in a dose-dependent manner in the FMRP-overexpressed cells, whereas the levels of the PA or NP proteins were comparable ( Fig. 3g,h ). These results were further confirmed with another RNP reconstitution system derived from the influenza A/Beijing/01/2009 (H1N1) virus (BJ09) ( Supplementary Fig. 5c–f ). Finally, we found that viral RNA synthesis in the RNP reconstitution system was greatly reduced in the cells treated with FMRP-specific siRNA, while re-expression of FMRP using an siRNA-resistant plasmid (FMRP SR ) ( Supplementary Fig. 5g,h ) restored the synthesis ( Fig. 3i ). Taken together, we conclude that FMRP is specifically involved in viral RNA synthesis by targeting the influenza A virus RNA synthesis machinery. FMRP interacts with NP and stimulates viral RNP assembly To further understand how FMRP targets influenza virus RNA synthesis machinery, we attempted to identify the interacting partner of FMRP within the RNP components. Flag-tagged FMRP was coexpressed with individual tandem affinity purification (TAP)-tagged RNP components (PB1-TAP, PB2-TAP, PA-TAP and TAP-NP). TAP-tagged proteins were then purified by IgG-Sepharose, and the association with FMRP was examined. FMRP was found to co-purify with TAP-NP, but not with the PB1-TAP or PB2-TAP ( Fig. 4a ). A faint band of Flag-tagged FMRP was observed with the PA-TAP purification sample. The FMRP and NP association was also confirmed in WSN virus-infected cells by immunoprecipitation ( Fig. 4b ), indicating that NP is the major binding partner of FMRP during influenza virus infection. 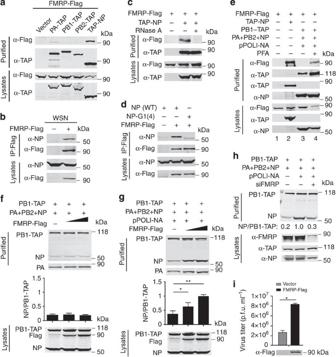Figure 4:FMRP interacts withNPin an RNA-dependent manner and stimulates viral RNP assembly and viral replication. (a) NP co-purifies with FMRP. The control vector, TAP-tagged PA, PB1, PB2 or NP expression constructs were individually transfected into 293T cells along with an FMRP-Flag plasmid. After 36 h, cells were lysed followed by TAP purification and western blot analyses. (b) FMRP associates with NP in WSN-infected cells. 293T cells were left untransfected or transfected with an FMRP-Flag plasmid. At 12 h.p.i. of WSN (MO1=1), cells were lysed and subjected to immunoprecipitation and western blot analyses. (c) FMRP interacts with NP in an RNA-dependent manner. 293T cells were transfected with TAP-NP or FMRP-Flag plasmids. Cell lysates were left untreated or were individually treated with RNase A for 1 h before being mixed together and TAP purified. (d) FMRP does not associate with the RNA-binding-deficient NP mutant. 293T cells were transfected with indicated plasmids and were analysed as described in (b). (e) FMRP transiently interacts with RNP. 293T cells were transfected with indicated plasmids. Cells were lysed and left untreated or treated with 0.5% PFA followed by TAP purification. (f) FMRP does not affect 4P association. 293T cells were transfected with PB1-TAP, PA, PB2 and NP plasmids along with increasing amounts of FMRP-Flag plasmids. Cells were then lysed followed by TAP purification (mean±s.d. of three independent experiments). (g) FMRP stimulates influenza virus RNP assembly. Cells were transfeced with indicated plasmids to reconstitute viral RNP and were analysed as described in (f) (mean±s.d. of three independent experiments, *P<0.05, **P<0.01, two-tailed Student’st-test). (h) Knockdown of FMRP reduces RNP assembly. 293T cells were transfected with control or FMRP-specific siRNA along with RNP reconstitution plasmids. Cells were then analysed as described in (f). (i) FMRP overexpression promotes virus production. Vero cells were transfected with a vector plasmid or FMRP-Flag plasmid. Cells were then infected with WSN (MOI=0.001). At 48 h.p.i., viral supernatants were harvested and then subjected to plaque assays (mean±s.d. of three independent experiments, *P<0.05, two-tailed Student’st-test). Figure 4: FMRP interacts with NP in an RNA-dependent manner and stimulates viral RNP assembly and viral replication. ( a ) NP co-purifies with FMRP. The control vector, TAP-tagged PA, PB1, PB2 or NP expression constructs were individually transfected into 293T cells along with an FMRP-Flag plasmid. After 36 h, cells were lysed followed by TAP purification and western blot analyses. ( b ) FMRP associates with NP in WSN-infected cells. 293T cells were left untransfected or transfected with an FMRP-Flag plasmid. At 12 h.p.i. of WSN (MO1=1), cells were lysed and subjected to immunoprecipitation and western blot analyses. ( c ) FMRP interacts with NP in an RNA-dependent manner. 293T cells were transfected with TAP-NP or FMRP-Flag plasmids. Cell lysates were left untreated or were individually treated with RNase A for 1 h before being mixed together and TAP purified. ( d ) FMRP does not associate with the RNA-binding-deficient NP mutant. 293T cells were transfected with indicated plasmids and were analysed as described in ( b ). ( e ) FMRP transiently interacts with RNP. 293T cells were transfected with indicated plasmids. Cells were lysed and left untreated or treated with 0.5% PFA followed by TAP purification. ( f ) FMRP does not affect 4P association. 293T cells were transfected with PB1-TAP, PA, PB2 and NP plasmids along with increasing amounts of FMRP-Flag plasmids. Cells were then lysed followed by TAP purification (mean±s.d. of three independent experiments). ( g ) FMRP stimulates influenza virus RNP assembly. Cells were transfeced with indicated plasmids to reconstitute viral RNP and were analysed as described in ( f ) (mean±s.d. of three independent experiments, * P <0.05, ** P <0.01, two-tailed Student’s t -test). ( h ) Knockdown of FMRP reduces RNP assembly. 293T cells were transfected with control or FMRP-specific siRNA along with RNP reconstitution plasmids. Cells were then analysed as described in ( f ). ( i ) FMRP overexpression promotes virus production. Vero cells were transfected with a vector plasmid or FMRP-Flag plasmid. Cells were then infected with WSN (MOI=0.001). At 48 h.p.i., viral supernatants were harvested and then subjected to plaque assays (mean±s.d. of three independent experiments, * P <0.05, two-tailed Student’s t -test). Full size image Both FMRP and NP are RNA-binding proteins. In addition, FMRP has been reported to interact with Tap/NXF1 in an RNA-dependent manner [22] . We therefore asked whether the interaction between FMRP and NP is mediated by RNAs. To test this, FMRP-Flag and TAP-NP were individually expressed, and the cell lysates were left untreated or treated with RNase A. On mixing the two pools of cell lysates, TAP purification of NP failed to bring down FMRP in the RNase A pretreated samples ( Fig. 4c ). Moreover, we found that RNase A treatment also disrupted the association between FMRP and NP in WSN virus-infected cells ( Supplementary Fig. 6a ). These results suggest that FMRP interacts with NP in an RNA-dependent manner. In support of these observations, the association between FMRP and an RNA-binding-deficient NP mutant [28] , [29] was substantially disrupted ( Fig. 4d ), confirming the role of RNAs in mediating the FMRP–NP association. Because NP is a major component of the RNP complex that serves as the functional unit for viral RNA synthesis, we next asked whether FMRP still associates with NP when it is already assembled as a component of RNP. To test this, NP was either expressed alone or in combination with PB1-TAP, PB2, PA and viral RNA that form a RNP complex. TAP purification revealed that FMRP could not be detected in the RNP sample in which a substantial amount of NP was present ( Fig. 4e , lane 3). Considering that FMRP is able to directly stimulate viral RNA synthesis that is catalysed by viral RNPs, we then speculated that FMRP might transiently interact with RNP. To test this, we treated the RNP sample with a crosslinking reagent (paraformaldehyde, PFA) before TAP purification to capture transient protein associations. Interestingly, the association of FMRP–RNP could now be detected ( Fig. 4e , lane 4), suggesting that FMRP can transiently associate with RNP. On the basis of the above observations that FMRP stimulates virus RNA synthesis in the RNP reconstitution system and that FMRP transiently interacts with RNP, we hypothesized that FMRP facilitates RNP assembly by RNA-mediated interactions with NP. To test this, we investigated the effects of FMRP overexpression on NP-associated interactions within the RNP complexes that are required for RNP assembly. NP interacts with itself, with RdRp and with viral RNA within the RNP complexes. We first examined the effect of FMRP on NP oligomerization and found that non-tagged NP associates with TAP-NP at similar levels with or without FMRP overexpression ( Supplementary Fig. 6b ), indicating that FMRP does not affect NP oligomerization. Then, using PB1-TAP as bait, we investigated the effects of FMRP overexpression on 3P (PB1, PB2 and PA) and 4P (3P+NP). We found that the levels of PA and NP did not change when FMRP was overexpressed ( Fig. 4f ; Supplementary Fig. 6c ), suggesting that FMRP does not exert its effect on the 3P or 4P complex assembly. In contrast, when viral RNAs were introduced into the 4P system that allowed formation of functional RNPs, FMRP stimulated the association of PB1-TAP with PA and NP in a dose-dependent manner ( Fig. 4g ). Moreover, PB1-TAP pulled down much less NP in the FMRP-knockdown cells compared with that in the control cells ( Fig. 4h ). Taken together, these results indicate that FMRP stimulates influenza virus RNP assembly. Since viral RNP assembly is one of the rate-limiting steps for influenza virus replication, we were then interested to test whether the FMRP overexpression could promote influenza virus production. We compared influenza virus growth in the FMRP-overexpressed Vero cells and in the control Vero cells. We found that influenza virus production is significantly higher with FMRP overexpression ( Fig. 4i ), indicating that FMRP promotes influenza virus replication. The KH2 domain is critical for stimulating RNP assembly To understand the functional significance of the RNA-dependent FMRP–NP association, we mapped the domain/motif of FMRP that is responsible for NP association. FMRP contains several motifs organized as NLS, KH1, KH2, nuclear export signal and RGG domains ( Fig. 5a ). Considering that the N terminus of FMRP is a conserved region for protein–protein interaction [30] and that NP–FMRP association is mediated by RNAs, we generated N-terminal FMRP truncation mutants (T1, T2 and T3) and FMRP RNA-binding domain deletion mutants (ΔKH1, ΔKH2 and ΔRGG) ( Fig. 5a ). We then examined the associations of NP with these mutants. While the N-terminal truncation mutants and the ΔKH1 and ΔRGG mutants bind efficiently to NP, the ΔKH2 mutant showed abrogated association with NP, suggesting an essential role of the KH2 domain in mediating FMRP–NP associations ( Fig. 5b ). 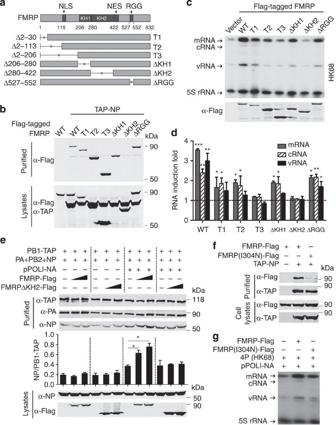Figure 5: FMRP KH2 domain mediates NP binding and is critical for stimulating RNA synthesis and viral RNP assembly. (a) Schematic of Flag-tagged FMRP truncation mutants. (b) FMRP interacts with NP via the KH2 domain. Flag-tagged FMRP truncation mutant plasmids were individually transfected into 293T cells together with TAP-NP plasmid. After 36 h, cell lysates were prepared followed by TAP purification and western blot analyses. (c) FMRP KH2 domain is critical for stimulating viral RNA synthesis. 293T cells were transfected with plasmids expressing the HK68 RNP reconstitution plasmids together with Flag-tagged full-length FMRP or FMRP truncation mutant plasmids. Total RNAs were extracted and levels of mRNA, cRNA and vRNA were detected by primer extension analyses. (d) Statistical analysis of viral RNAs in (c). Values of viral RNAs in cells transfected with full-length FMRP or FMRP mutants were standardized to the 5S rRNA level and then normalized to levels of viral RNAs in cells transfected with a control vector (mean±s.d. of three independent experiments, *P<0.05, **P<0.01 and ***P<0.001, two-tailed Student’st-test). (e) The FMRP KH2 domain is critical for stimulating viral RNP assembly. 293T cells were transfected with plasmids expressing PB1-TAP, PA, PB2 and NP, with or without the viral RNA expression plasmid, along with increasing amounts of the FMRP or FMRP-ΔKH2 plasmid. After 36 h, cell lysates were prepared followed by TAP purification and western blot analyses (mean±s.d. of three independent experiments, *P<0.05, two-tailed Student’st-test). (f) A point mutation (I304N) in the KH2 domain of FMRP disrupts FMRP–NP association. 293T cells were transfected with Flag-tagged WT FMRP or FMRP I304N mutant expression plasmids together with TAP-NP. After 36 h, cell lysates were prepared followed by TAP purification and western blot analyses. (g) The FMRP I304N mutant is defective in stimulating viral RNA synthesis. 293T cells were transfected with Flag-tagged WT FMRP or FMRP (I304N) plasmids together with the HK68 RNP reconstitution system. Total RNAs were prepared and analysed as indicated in (c). Figure 5: FMRP KH2 domain mediates NP binding and is critical for stimulating RNA synthesis and viral RNP assembly. ( a ) Schematic of Flag-tagged FMRP truncation mutants. ( b ) FMRP interacts with NP via the KH2 domain. Flag-tagged FMRP truncation mutant plasmids were individually transfected into 293T cells together with TAP-NP plasmid. After 36 h, cell lysates were prepared followed by TAP purification and western blot analyses. ( c ) FMRP KH2 domain is critical for stimulating viral RNA synthesis. 293T cells were transfected with plasmids expressing the HK68 RNP reconstitution plasmids together with Flag-tagged full-length FMRP or FMRP truncation mutant plasmids. Total RNAs were extracted and levels of mRNA, cRNA and vRNA were detected by primer extension analyses. ( d ) Statistical analysis of viral RNAs in ( c ). Values of viral RNAs in cells transfected with full-length FMRP or FMRP mutants were standardized to the 5S rRNA level and then normalized to levels of viral RNAs in cells transfected with a control vector (mean±s.d. of three independent experiments, * P <0.05, ** P <0.01 and *** P <0.001, two-tailed Student’s t -test). ( e ) The FMRP KH2 domain is critical for stimulating viral RNP assembly. 293T cells were transfected with plasmids expressing PB1-TAP, PA, PB2 and NP, with or without the viral RNA expression plasmid, along with increasing amounts of the FMRP or FMRP-ΔKH2 plasmid. After 36 h, cell lysates were prepared followed by TAP purification and western blot analyses (mean±s.d. of three independent experiments, * P <0.05, two-tailed Student’s t -test). ( f ) A point mutation (I304N) in the KH2 domain of FMRP disrupts FMRP–NP association. 293T cells were transfected with Flag-tagged WT FMRP or FMRP I304N mutant expression plasmids together with TAP-NP. After 36 h, cell lysates were prepared followed by TAP purification and western blot analyses. ( g ) The FMRP I304N mutant is defective in stimulating viral RNA synthesis. 293T cells were transfected with Flag-tagged WT FMRP or FMRP (I304N) plasmids together with the HK68 RNP reconstitution system. Total RNAs were prepared and analysed as indicated in ( c ). Full size image We next tested the effects of these FMRP mutants in stimulating viral RNA synthesis in the HK68 and BJ09 RNP reconstitution systems. In line with the interaction data, overexpression of the ΔKH2 mutant failed to stimulate viral RNA synthesis, while other truncation mutants stimulated RNA synthesis, albeit at different extents ( Fig. 5c,d ; Supplementary Fig. 7a,b ). We noticed that the T3 mutant also showed little stimulating effects. This can be explained by the fact that the T3 mutant, which is devoid of the NLS of FMRP, failed to enter the nucleus ( Supplementary Fig. 7c ) where FMRP carries out its function. Taken together, these data suggest that the KH2 domain of FMRP plays a crucial role in mediating NP interaction and stimulating viral RNA synthesis, though the intact protein is required for full activity. To further study the role of the KH2 domain, we tested the effect of the ΔKH2 mutant on stimulating RNP assembly. Although overexpression of the full-length FMRP stimulated PA/NP association with PB1 in a dose-dependent manner, overexpression of the ΔKH2 FMRP mutant failed to do so ( Fig. 5e ). Neither the ΔKH2 FMRP mutant nor the full-length FMRP had an effect on the 4P system ( Fig. 5e ). These results confirmed that the KH2 domain of FMRP plays a key role in stimulating influenza virus RNP assembly by mediating an FMRP–NP association. The X-ray crystal structure of the KH1–KH2 domains of human FMRP suggests that the I304N mutation in the KH2 domain disrupts the normal folding and the structure of the KH1–KH2 peptide [31] . In addition, the I304N mutation associates with a particularly severe incidence of Fragile X syndrome [26] . In our system, the FMRP I304N mutation significantly disrupted the interaction between FMRP and NP ( Fig. 5f ) and the stimulating effect of FMRP on viral RNA/protein synthesis and viral RNP assembly ( Fig. 5g ; Supplementary Fig. 7d,e ). These results indicate that functional FMRP is critical for stimulating influenza virus RNP assembly and subsequent RNA synthesis. FMRP knockdown leads to nuclear retention of RNP components It is known that vRNPs are assembled in the nucleus and exported to the cytosol as a complex [9] . Thus, it can be speculated that RNP components might be retained in the nucleus if the RNP assembly is attenuated. Indeed, we initially observed that the knockdown of FMRP led to nuclear retention of NP in infected cells. Therefore, we then examined whether other RNP components, in addition to NP, were retained in the nucleus of FMRP-knockdown cells in the late stages of virus replication. The in situ hybridization assay showed that vRNAs, a key component of vRNP, were largely retained in the nucleus on FMRP knockdown. In contrast, viral mRNAs, which are transported to the cytosol independently of vRNP [32] , were sufficiently exported ( Fig. 6a,b ; Supplementary Fig. 8a ). Furthermore, confocal microscopy analysis revealed that PA, another vRNP component, accumulated in the nucleus when FMRP was knocked down ( Fig. 6c,e ), while the distribution of viral nuclear export protein (NEP) was not substantially affected ( Fig. 6d,e , also see Discussion). Moreover, siRNA-resistant WT FMRP or the I304N mutant (FMRP SR , FMRP(I304N) SR ) was reconstituted in the FMRP-knockdown cells, and cellular distributions of NP and PA on viral infection were examined. We found that WT FMRP could substantially restore nuclear export of both NP and PA, while the I304N mutant failed to do so ( Supplementary Fig. 8b–d ). Together, these results suggest that FMRP is required for nuclear export of the RNP components. This is likely due to its role in RNP assembly as described above. 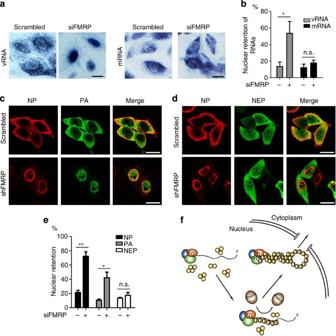Figure 6: FMRP knockdown leads to nuclear retention of RNP components. (a) FMRP knockdown leads to nuclear retention of vRNAs but does not affect viral mRNA trafficking. A549 cells were transfected with control or FMRP-specific siRNAs. After 48 h, cells were infected with PR8 virus for 9 h and subjected toin situhybridization assays using vRNA-specific (left) or mRNA-specific (right) probes against theM1gene. Scale bar, 10 μm. (b) Statistical analysis of RNA distribution in (a) (mean±s.d. of two independent experiments, *P<0.05, n.s., not significant, two-tailed Student’st-test). (c,d) FMRP knockdown impedes PA nuclear export but does not affect NEP nuclear export. Control or FMRP-knockdown cells were infected with PR8 virus for 9 h followed by immunofluorescence analysis with indicated antibodies. Scale bar, 10 μm. (e) Statistical analysis of viral protein distribution in (c) and (d). Quantitative analyses were calculated by ratios of NP nuclear-retained cells/total infected cells (mean±s.d. of three independent experiments, *P<0.05, **P<0.01, n.s., not significant, two-tailed Student’st-test). (f) Proposed model for the role of FMRP during influenza virus replication. Figure 6: FMRP knockdown leads to nuclear retention of RNP components. ( a ) FMRP knockdown leads to nuclear retention of vRNAs but does not affect viral mRNA trafficking. A549 cells were transfected with control or FMRP-specific siRNAs. After 48 h, cells were infected with PR8 virus for 9 h and subjected to in situ hybridization assays using vRNA-specific (left) or mRNA-specific (right) probes against the M1 gene. Scale bar, 10 μm. ( b ) Statistical analysis of RNA distribution in ( a ) (mean±s.d. of two independent experiments, * P <0.05, n.s., not significant, two-tailed Student’s t -test). ( c , d ) FMRP knockdown impedes PA nuclear export but does not affect NEP nuclear export. Control or FMRP-knockdown cells were infected with PR8 virus for 9 h followed by immunofluorescence analysis with indicated antibodies. Scale bar, 10 μm. ( e ) Statistical analysis of viral protein distribution in ( c ) and ( d ). Quantitative analyses were calculated by ratios of NP nuclear-retained cells/total infected cells (mean±s.d. of three independent experiments, * P <0.05, ** P <0.01, n.s., not significant, two-tailed Student’s t -test). ( f ) Proposed model for the role of FMRP during influenza virus replication. Full size image The interplay between the influenza virus and host is a dynamic process that determines the pathogenicity and host specificity of the virus. Several independent genome-wide RNAi screens with different approaches have been conducted in the last couple of years and have identified over a thousand human genes that could be associated with influenza virus infection [1] , [2] , [3] , [4] , [5] , [6] . Here we performed a cellular transcriptional-based siRNA screen and found that among 300 viral inducible genes, 52 could potentially regulate influenza virus replication. Forty of these genes have not been reported in the previous screens, in which the antiviral host factor HERC5, has been recently shown to attenuate influenza virus replication [33] . Among the reported 12 genes, B2M, IFIT5 and RPS4X have been identified in other two independent screens, suggesting that these genes are promising candidates for further investigation. Notably, there is a strong overlap between results from Shapira et al. [5] and ours. This could result from similar screen strategies that are based on transcriptional profiling. In addition, functional classification analysis revealed that 6 of the 52 identified genes, including FMR1 , have RNA-binding activities. Considering RNA-binding activities of host factors are critical in facilitating influenza virus RNA transcription, replication and trafficking, it is possible that these host factors could be involved in viral RNA biogenesis. Further functional studies of these host factors will help to unveil influenza virus and host interplays. In this report, we identified FMRP as a positive regulator of influenza virus replication by an siRNA screen. We demonstrated that FMRP acts as a transient stimulator of influenza virus RNP assembly through RNA-mediated interaction with NP. Further analyses revealed that the KH2 domain of FMRP plays a critical role in the FMRP–NP association and vRNP assembly. We propose that FMRP is used by the influenza virus for its efficient replication in the host, given that FMRP is expressed in epithelial cells including the ciliated columnar epithelium lining of the airways [34] that are the sites of influenza virus replication, and that FMRP is upregulated on influenza virus infection. Because FMRP stimulates influenza virus production, FMRP-stable overexpression cell lines could be used for influenza vaccine production as a means to increase virus yield. Taking advantage of the microscopy-based siRNA screen, we initially observed that knockdown of the FMR1 gene led to nuclear retention of NP during viral infection. Subsequently, we found that other RNP components, including PA and vRNA, were also retained in the nucleus on FMRP knockdown. Considering that vRNP components are exported to the cytosol as a complex and that FMRP exerts its function in viral RNP assembly, we inferred that nuclear accumulation of RNP components is a secondary effect of the insufficient assembly of RNPs. In support of this, reconstitution of WT FMRP expression restored NP and PA nuclear export, whereas the I304N mutant, which maintained its ability in nucleocytoplasmic shuttling [35] but lost its function in RNP assembly, failed to do so. We noticed that knockdown of FMRP had little effect on viral mRNA and NEP distribution ( Fig. 6a,b,d,e ). This can be explained by the fact that mRNA and NEP could conduct nuclear export independent of vRNP [32] , [36] . Overall, our results suggest that FMRP is specifically involved in vRNP biogenesis of the influenza A virus ( Fig. 6f ). Research of FMRP from the past two decades led to the understanding of its functions in neuron cells where it regulates mRNA transport and translational control [23] , [24] , [25] . Here, in the context of the influenza virus infection, we found that FMRP is not required for viral mRNA nuclear export but is required for vRNP assembly, suggesting a novel role of FMRP. Our observations favour that FMRP plays a role in vRNP assembly via KH2 domain-mediated FMRP–NP association that is dependent on RNAs. Structural studies of the KH2 domain in Nova-1 and Mycobacterium tuberculosis NusA suggest that the KH2 domain associates with nucleotide bases [37] , [38] . The crystal structure of a trimeric ring-like NP complex reveals that NP monomers possess a positively charged RNA-binding groove [28] , [39] , which should be in contact with the phosphate-sugar backbone of the RNA. The RNA-binding properties of these proteins may allow formation of a sandwich-like NP–RNA–FMRP structure, in which NP binds to the backbone of the RNA from one side and FMRP binds to the nucleotide bases of the RNA from the other side. Targeting this NP–RNA–FMRP association may provide a novel option for drug development against influenza virus infection. Viruses and cells Influenza A/WSN/33 and A/PR/8/34 viruses were kindly provided by Dr Ervin Fodor (University of Oxford, UK). Influenza A/Anhui/1/2013 virus (H7N9) was kindly provided by Dr Yuelong Shu (Chinese Center for Disease Control and Prevention). The human lung carcinoma cell line A549, Madin–Darby canine kidney (MDCK), 293T and HeLa cells were purchased from the American Type Culture Collection (ATCC, Manassas, VA) and were maintained in Dulbecco’s modified Eagle’s medium (Invitrogen, Carlsbad, CA) supplemented with 10% fetal bovine serum (HyClone, Logan, UT), 100 U ml −1 penicillin and 100 μg ml −1 streptomycin at 37 °C. Plasmids and antibodies The full-length Flag-tagged FMRP expression plasmid was purchased from Origene (Rockville, MD, USA). The FMRP truncations and point mutations were generated using a QuikChange Site-Directed Mutagenesis kit (Stratagene, La Jolla, CA). The pcDNA plasmids of the RNP reconstitution system of influenza A/HongKong/1/1968 (H3N2) were constructed from plasmids kindly provided by Dr Earl G. Brown (University of Ottawa, Canada). The pcDNA plasmids of RNP reconstitution system of influenza A/Beijing/01/2009 (H1N1) were constructed by RT–PCR amplification from a virus isolated from a hospitalized patient in Beijing. The primers used in reverse transcription were a mixture of two primers 5′-AGCAAAAGCGGA-3′ and 5′-AGCGAAAGCGGA-3′ corresponding to natural viral RNA promoter region at the 3′ end. The TAP-tagged or non-tagged pcDNA plasmids encoding PB1, PB2, PA, NP, NP-G1(4) and two viral RNA expressing plasmids pPOLI-NA-RT, pPOLI-HA-RT derived from influenza A/WSN/33 have been described previously [16] , [29] . Rabbit anti-Lamin A (1:2,000, L1293), rabbit anti-GAPDH (1:4,000, G9545), mouse monoclonal anti-β-actin (1:4,000, A5441) and mouse monoclonal anti-Flag M2 (1:4,000, F3165) were purchased from Sigma-Aldrich. The mouse monoclonal anti-influenza NP (1:2,000, MAB8251) and anti-FMRP (1:1000, MAB2160) were purchased from Millipore (Temecula, CA). Rabbit anti-TAP (1:1,000, sc-25768) was purchased from Santa Cruz Biotechnology (Santa Cruz, CA). Rabbit polyclonal anti-PA (1:1,000) was kindly provided by Dr Ervin Fodor. Microarray analysis and siRNA screen For microarray analysis, A549 cells were infected with influenza A/PR/8/34 virus at a multiplicity of infection (MOI) of 0.5. Total RNA was then extracted at 4, 12, 24 h and 48 h.p.i. and subjected to global gene expression analysis by microarray chips (Capitalbio human genome oligo array service). For the siRNA screen, a siRNA library specific for the upregulated host genes determined by microarray analysis were designed and synthesized by Dharmacon (Boulder, CO) (orders 193155, 193158, 193161 and 193162). A549 cells in 96-well plates were transfected with siRNAs (50 nM) using Dharmafect 1 reagent (Dharmacon, Boulder, CO) for 72 h and were then infected with PR8 virus at an MOI of 0.1 or 0.5. At 16 h.p.i., cells were fixed and stained with an influenza NP-specific antibody. Images were acquired using a fluorescence microscope and then analysed by the Image-Pro Plus software. RNA interference Cells were transfected with siRNAs at 50 nM for indicated times. The following sequences were targeted for FMR1 (5′→3′): #1: 5′-CCAAAGAGGCGGCACAUAA-3′; #2: 5′-AAAGCUAUGUGACUGAUGA-3′; #3: 5′-CAGCUUGCCUCGAGAUUUC-3′. Lentivirus expressing FMRP-specific short-hairpin RNA was generated by the GenePharma Company (Shanghai). Briefly, two complementary oligonucleotides with Bam H1 and Eco RI endonuclease sites at each end were synthesized, annealed and cloned into a HIV-based lentiviral expression vector (LV3-pGLV-H1-GFP/PURO, GenePharma, Shanghai) to express a hairpin transcript (5′-GCAGCTTGCCTCGAGATATCTCAAGAGGATATCTCGAGGCAAGCTGCTT-3′). The lentiviral particles were then produced by cotransfecting the short-hairpin RNA expression plasmids with packaging plasmids into 293 packaging cells. After 72 h, viruses were collected and titred. To generate FMRP-stable knockdown or control cell lines, 293T or HeLa cells were infected with the lentiviral particles and selected with puromycin (1 μg ml −1 ) for 3 weeks. TCID 50 assay and plaque assay For the WSN and the recombinant Newcastle disease virus, TCID 50 assays were performed in MDCK cells and 293T cells, respectively, according to a protocol described in http://www.who.int/csr/resources/publications/influenza/en/whocdscsrncs20025rev.pdf . Data were analysed according to the Reed and Muench method [40] . To determine the plaque-forming unit, viral supernatants were collected and plaque titres were determined by the plaque assay [41] . Briefly, monolayer MDCK cells in 3.5-cm dishes were incubated with serial dilutions (10 times) of viral supernatants in 0.1 ml at room temperature (RT) for 1 h with swirling every 15 min. Two millilitres of 1% agarose with 0.25% fetal bovine serum were then added to the cells and left at RT until it set. Then the dishes were turned upside down and incubated at 37 °C. At 72 h post infection, the agarose layer was removed and the plaques were visualized with 0.1% crystal violet solution. Animal experiments The animal experiments were performed according to the protocols approved by the Institute of Animal Use and Care Committee of the Institute of Laboratory Animal Science, Peking Union Medical College (ILAS-PC-2010-002). Six-week-old male WT ( n =11) and FMR1 -gene knockout (FMRP −/− ) ( n =23) mice in the FVB.129P2(B6)-Fmr1tm1Cgr/J strain background were kindly provided by Dr B. Oostra. Mice were genotyped and the lack or presence of the Fmr1 gene was confirmed by PCR. WT and FMRP −/− animals were anaesthetized with pentobarbital and inoculated intranasally with 10 4 TCID 50 of the A/PR/8/34 influenza virus in a volume of 50 μl diluted in phosphate-buffered saline (PBS). Control groups ( n =8) received PBS only. The virus inoculation is a blind procedure performed by a well-trained professional who routinely conducts mouse virus infection experiments and is not aware of the mouse genotypes for infection. Animals were observed for 2 weeks, and weight loss and other signs of disease were assessed. For detection of viral titres, three mice per group were euthanized on days 3 and 6 p.i. Virus titres were determined by plaque assays in MDCK cells. For histopathologic analysis, lungs were removed on day 3 p.i. and fixed with 4 % PFA. Lung samples were embedded in paraffin and cut into 4-μm-thick sections, followed by staining with haematoxylin and eosin (H&E). For the lung histology score, images were evaluated by an investigator in a blinded manner following a standardized score system as previously described [42] . For immunohistochemistry, lung tissue sections were quenched in 3% H 2 O 2 and then pretreated with proteinase K for 15 min. Slides were blocked for 30 min, rinsed with Tris-buffered saline with Tween 20 (TBST) and incubated with anti-NP (MAB8251, Millipore) at a 1:500 dilution for 2 h. The sections were then incubated with polymer HRP for 15 min, reacted with the chromogen diaminobenzidine and counterstained with Gill’s haematoxylin stain. TAP purification and immunoprecipitation TAP purification has been described previously [43] . For immunoprecipitation, transfected cells were lysed with radioimmunoprecipitation assay buffer. Lysates were incubated overnight at 4 °C with various antibodies indicated, followed by an incubation with protein A/G agarose beads (Santa Cruz Biotechnology) for 2 h at 4 °C. After extensive washes, immunocomplexes captured on protein A/G agarose beads were then subjected to western blot analysis. For crosslinking experiments, transfected cells were washed in PBS and then treated with 0.5% PFA at 37 °C. After 15 min, the reaction was terminated by adding glycine to 125 mM for 5 min at RT. The cells were then treated as described previously [44] and subjected to TAP purification. Western blot and primer extension analyses Samples were separated by SDS–PAGE and immunoblotted with indicated primary antibodies and IRDye Secondary Antibodies (LI-COR Biosciences, Lincoln, NE). Protein expression levels were detected using the Odyssey Infrared Imaging System (LI-COR Biosciences). The relative protein expression level was analysed using the integrated software of the Odyssey system. The levels of three viral RNA species (mRNA, cRNA and vRNA) were determined by primer extension analysis with two 32 P-labelledNA-specific primers: 5′-TGGACTAGTGGGAGCATCAT-3′ (to detect vRNA) and 5′-TCCAGTATGGTTTTGATTTCCG-3′ (to detect mRNA and cRNA). Transcription products were analysed on 6% polyacrylamide gels containing 7 M urea in TBE buffer, detected by autoradiography and quantified by phosphorimage analysis [45] . Full western blots and autoradiographs are provided in Supplementary Fig. 9 . Indirect immunofluorescence assay A549 or HeLa cells either infected or mock-infected with influenza A virus were fixed in 4% PFA and permeabilized with PBS containing 0.5% Triton X-100, followed by blocking with PBS containing 0.1% Tween and 5% bovine serum albumin. The cells were then incubated with anti-influenza NP antibody (1:500) at 4 °C overnight. After extensive washes, cells were incubated with anti-mouse DyLight 594-conjugated antibody (1:500; Zhongshanjinqiao Biotech Co., Beijing, China) for 1 h at RT, and cell nuclei were labelled with 4′,6-diamidino-2-phenylindole (DAPI) reagent (Sigma-Aldrich). Fluorescence images were obtained by a Leica TCS SP5 laser scanning confocal microscope. Nuclear and cytoplasmic protein fractionation Cells were harvested and washed with pre-cold PBS. Then, according to the manufacturer’s instructions, nuclear and cytoplasmic fractions were separated using the NE-PER Nuclear and Cytoplasmic Extraction Kit (Thermo Fisher, Rockford, IL). In situ hybridization assay The probes for detecting viral mRNAs and vRNAs ( M1 gene) were prepared as previously described [46] . Briefly, to generate the probe for detecting vRNAs, we linearized pcDNA-M1 plasmid and then used it as a template for in vitro transcription using the TranscriptAid T7 High Yield Transcription Kit (Thermo Fisher, USA). To generate the probe for detecting viral mRNAs, we constructed a pCDNA3.1-rM1 plasmid encoding the reverse complementary sequence of M1 and used it as a template for in vitro transcription. The in vitro transcription was carried out according to the manufacturer’s manual with digoxigenin-labelled UTP (Roche, UK) added in the reaction. The RNA transcripts were purified by isopropanol precipitation and dissolved in RNase-free water. For in situ hybridization analysis, influenza A virus-infected A549 cells were fixed with 4% PFA and 5% acetic acid in 0.15 M NaCl at −20 °C for 17 min. After washing three times with PBS, cells were permeabilized with 0.01% pepsin (pH 2.0) at 37 °C for 5 min. Cells were washed again, post-fixed using 4% PFA in PBS at −20 °C for 10 min and washed again with PBS. Cells were then pre-hybridized using a pre-hybridization solution (60% formamide, 0.3 M sodium chloride, 30 mM sodium citrate (pH 7.0), 10 mM EDTA (pH 8), 35 mM NaH 2 PO 4 , 5% dextran sulphate, 250 ng ml −1 tRNA) at 37 °C for 1 h. During this period, digoxigenin-labelled ribonucleotide probes were heated to 85 °C for 5 min and placed on ice for another 5 min. Then, cells were incubated with hybridization solution (0.7 ng μl −1 mRNA or 1ng μl −1 vRNA probe against the influenza virus M1 gene and 20 U ml −1 RNase inhibitor in pre-hybridization solution) at 37 °C for at least 16 h. Cells were then washed three times for 15 min at 37 °C and two times for 5 min at RT with 0.2 × SSC. Further washes were conducted in buffer B1 (0.1 M Tris–HCl (pH 7.4) and 0.15 M NaCl) for 5 min, followed by the addition of blocking solution (10% goat serum in buffer B1) for 1 h at RT. Then, blocking solution was replaced with anti-Dig-alkaline phosphatase (1:5,000, Sigma) in blocking solution and the samples were incubated at 4 °C overnight. After washing three times with buffer B1, the samples were equilibrated twice with buffer B2 (0.1 M Tris–HCl (pH 9.5), 0.15 M NaCl, 0.05 M MgCl 2 and 0.1% Tween-20) for 5 min. Samples were visualized using NBT/BCIP in buffer B2 and images were acquired with a Nikon microscope. Statistical analysis Student’s t -test was used for two-group comparisons. The * P -value <0.05, ** P -value <0.01 and *** P -value <0.001 were considered significant. How to cite this article: Zhou, Z. et al. Fragile X mental retardation protein stimulates ribonucleoprotein assembly of influenza A virus. Nat. Commun. 5:3259 doi: 10.1038/ncomms4259 (2014).